Characterizing the genetic basis of methylome diversity in histologically normal human lung tissue The genetic regulation of the human epigenome is not fully appreciated. Here we describe the effects of genetic variants on the DNA methylome in human lung based on methylation-quantitative trait loci (meQTL) analyses. We report 34,304 cis - and 585 trans -meQTLs, a genetic–epigenetic interaction of surprising magnitude, including a regulatory hotspot. These findings are replicated in both breast and kidney tissues and show distinct patterns: cis -meQTLs mostly localize to CpG sites outside of genes, promoters and CpG islands (CGIs), while trans -meQTLs are over-represented in promoter CGIs. meQTL SNPs are enriched in CTCF-binding sites, DNaseI hypersensitivity regions and histone marks. Importantly, four of the five established lung cancer risk loci in European ancestry are cis- meQTLs and, in aggregate, cis -meQTLs are enriched for lung cancer risk in a genome-wide analysis of 11,587 subjects. Thus, inherited genetic variation may affect lung carcinogenesis by regulating the human methylome. DNA methylation plays a central role in epigenetic regulation. Twin studies have suggested that DNA methylation at specific CpG sites can be heritable [1] , [2] ; however, the genetic effects on DNA methylation have been investigated only in brain tissues [3] , [4] , adipose tissues [5] , [6] and lymphoblastoid cell lines [7] . Most studies were based on the Illumina HumanMethylation27 array, which has a low density and mainly focuses on CpG sites mapping to gene promoter regions. While the functional role of DNA methylation in non-promoter or non-CpG Island (CGI) regions remains largely unknown, evidence shows roles in regulating gene splicing [8] and alternative promoters [9] , silencing of intragenic repetitive DNA sequences [10] , and predisposing to germline and somatic mutations that could contribute to cancer development [11] , [12] . Notably, a recent study [13] suggests that most DNA methylation alterations in colon cancer occur outside of promoters or CGIs, in so called CpG island shores and shelves, and the Cancer Genome Project has reported high mutation rates in CpG regions outside CGI in multiple cancers [14] . Although expression QTLs (eQTLs) have been extensively studied in different cell lines and tissues [15] , the minimal overlap observed between cis -acting meQTLs and eQTLs (≈5–10%) [3] , [4] , [7] emphasizes the necessity of mapping meQTLs that may function independently of nearby gene expression. This might reveal novel mechanisms for genetic effects on cancer risk, particularly since many of the established cancer susceptibility SNPs map to non-genic regions. Lung diseases constitute a significant public health burden. About 10 million Americans had chronic obstructive pulmonary disease in 2012 (ref. 16) [16] and lung cancer continues to be the leading cancer-related cause of mortality worldwide [17] . To provide functional annotation of SNPs, particularly those relevant to lung diseases and traits, we systematically mapped meQTLs in 210 histologically normal human lung tissues using Illumina Infinium HumanMethylation450 BeadChip arrays, which provide a comprehensive platform to interrogate the DNA methylation status of 485,512 cytosine targets with excellent coverage in both promoter and non-promoter regions ( Fig. 1a ), CGI and non-CGI regions ( Fig. 1b ) and gene and non-gene regions. Thus, our study enables the characterization of genetic effects across the methylome in unprecedented detail. Moreover, since DNA methylation exhibits tissue-specific features [18] , we investigated whether similar meQTLs could be identified in other tissues. 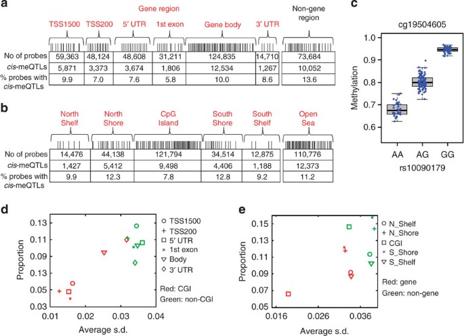Figure 1:cis-meQTL structural characteristics. (a) Distribution of CpG probes and correspondingcis-meQTL numbers and proportions in gene and non-gene regions. meQTLs were detected based on EAGLE lung normal tissue samples (n=210). (b) Distribution of CpG probes and correspondingcis-meQTL numbers and proportions in CpG islands (CGIs), shores (<2 kb from the boundary of CGI), shelves (2–4 kb from the boundary of CGI) and the remaining region or ‘open sea’. (c) The strongestcis-association is between SNP rs10090179 and CpG probe cg19504605.P=1.5 × 10−73,t-test. The SNP explains 79.8% of the phenotypic variance. The box plots show the distribution of the methylation levels in each genotype category with error bars representing the 25 and 75% quantiles. (d,e) Thexcoordinate is the average s.d. of methylation levels for CpG probes in each category. Theycoordinate is the proportion of CpG probes detected withcis-meQTLs. The proportion of methylation probes detected withcis-meQTLs varied across categories, ranging from 4.0% for CGIs in 1st exons to 15.7% for south shores in non-gene regions. Figure 1: cis -meQTL structural characteristics. ( a ) Distribution of CpG probes and corresponding cis -meQTL numbers and proportions in gene and non-gene regions. meQTLs were detected based on EAGLE lung normal tissue samples ( n =210). ( b ) Distribution of CpG probes and corresponding cis -meQTL numbers and proportions in CpG islands (CGIs), shores (<2 kb from the boundary of CGI), shelves (2–4 kb from the boundary of CGI) and the remaining region or ‘open sea’. ( c ) The strongest cis -association is between SNP rs10090179 and CpG probe cg19504605. P =1.5 × 10 −73 , t -test. The SNP explains 79.8% of the phenotypic variance. The box plots show the distribution of the methylation levels in each genotype category with error bars representing the 25 and 75% quantiles. ( d , e ) The x coordinate is the average s.d. of methylation levels for CpG probes in each category. The y coordinate is the proportion of CpG probes detected with cis -meQTLs. The proportion of methylation probes detected with cis -meQTLs varied across categories, ranging from 4.0% for CGIs in 1st exons to 15.7% for south shores in non-gene regions. Full size image Identification of cis -acting meQTLs We profiled DNA methylation for 244 fresh-frozen histologically normal lung samples from non-small cell lung cancer (NSCLC) patients from the Environment and Genetics in Lung cancer Etiology (EAGLE) study [19] . A subset of 210 tissue samples that passed quality control and had germline genotype data from blood samples [20] was used for meQTL analysis. The analysis was restricted to 338,456 autosomal CpG probes after excluding those annotated in repetitive genomic regions or that harboured genetic variants. The distribution of methylation levels differed strongly across distinct types of genomic regions ( Supplementary Fig. 1a,b ). Consistent with previous studies [21] , CpG sites in promoter or CGI regions were largely unmethylated while those in other regions were largely methylated ( Supplementary Fig. 1a,b ). We performed cis -meQTL analysis for each methylation trait by searching for SNPs within 500 kb of the target CpG-site in each direction (1 Mb overall). The genetic association was tested under an additive model between each SNP and each normalized methylation probe, adjusting for sex, age, plate, population stratification and methylation-based principal component analysis (PCA) scores. Controlling FDR at 5% ( P =4.0 × 10 −5 ), we detected cis -meQTLs for 34,304 (10.1% of 338,456) CpG probes ( Supplementary Table 1 ), mapping to 9,330 genes. A more stringent threshold ( P =6.0 × 10 −6 ) at FDR=1% detected cis -meQTLs for 27,043 CpG probes, mapping to 8,479 genes. Moreover, with a 200-kb window (100 kb from both sides) instead of a 1-Mb window we detected 40,650 cis -meQTLs ( P =2.0 × 10 −4 ), controlling for FDR=5%. The methylation distribution in CpG sites detected with meQTLs differed substantially from those without meQTLs ( Supplementary Fig. 1a,b ). The peak SNPs were equally distributed on either side of the target CpG sites with a median distance (Δ) of 11.8 kb. The proportion of explained phenotypic variance ( h 2 ) ranged from 7.7 to 79.8% ( Supplementary Fig. 1c ) and inversely depended on Δ ( Supplementary Fig. 1d ). We detected strong cis -meQTLs for DNMT1 , a gene known for establishment and regulation of tissue-specific patterns of methylated cytosine residues, and for DNMT3A/B , two genes involved in de novo methylation in mammals, but not for MTHFR , which affects global methylation ( Supplementary Fig. 1e ). The likelihood of detecting cis -meQTLs varied across CpG regions and strongly depended on the variability of the methylation levels ( Fig. 1d,e ). CpG probes in non-CGI regions were twice as likely to harbour cis -meQTLs than CpG probes in CGI regions (11.5 versus 4.8%, t -test P <10 −100 ); similarly, CpG probes located in CGI of non-gene regions were twice as likely to harbour cis meQTL than those in gene regions (14.6 versus 6.6%, t -test P <10 −100 ). To verify the cis -meQTLs, we analysed data from The Cancer Genome Atlas (TCGA) [22] NSCLC patients ( n =65) for whom both DNA methylation data from llumina HumanMethylation450 BeadChip of histologically normal lung tissue and germline genotypes from Affymetrix Genome-Wide Human SNP Array 6.0 were available. Genetic associations were tested using the imputed genotypic dosages. EAGLE findings were strongly replicated in TCGA lung data: for the 34,304 associations detected in EAGLE, 32,128 (93.7%) had the same direction and 22,441 (65.4%) had FDR<0.05 based on single-sided P -values ( Table 1 ). Table 1 Replication of EAGLE lung meQTLs in TCGA histologically normal tissue samples. Full size table For 34,304 CpG probes detected with cis -meQTLs, we searched for secondary independently associated SNPs in cis regions by conditioning on the primary cis -meQTL SNPs. We detected secondary cis -meQTL SNPs for 3,546 CpG probes (FDR=5%, P =4 × 10 −5 ), 61.5% of which were replicated in TCGA lung data. Identification of trans -acting meQTLs Identification of trans -meQTLs was performed by searching for SNPs that were on different chromosomes from the target CpG sites or on the same chromosome but >500 kb away. We detected 615 CpG probes with trans -meQTLs (FDR=5%, P =2.5 × 10 −10 ), including 438 interchromosomal and 177 intrachromosomal trans -meQTLs. Among 177 intrachromosomal trans associations, 30 lost significance after conditioning on the corresponding cis -regulating SNPs, suggesting that these trans associations were caused by cis -acting regulations through long-range linkage disequilibrium (LD). Thus, we detected 585 traits with ‘true’ trans -meQTLs ( Fig. 2a ), mapping to 373 genes. The number of trans -meQTLs was reduced to 500 if controlling for FDR=1% ( P =4.0 × 10 −11 ). We replicated 79.8% of the 585 trans associations in TCGA lung data. Interestingly, trans -meQTLs were strongly enriched in CGI sites, in contrast to the observation that cis -meQTLs were strongly enriched in non-CGI sites ( Fig. 2b ). CpG dinucleotides in 3′ UTR regions, where microRNA target sites are typically located, showed an opposite trend in both cis - and trans -meQTLs ( Fig. 2b ). 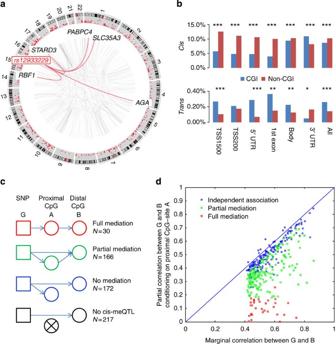Figure 2:trans-meQTL structural characteristics. (a) Circos plot fortrans-meQTLs. The outer rim shows the log10P-values Manhattan plots oftrans-meQTL associations. The innermost network depicts spokes between alltrans-meQTL SNPs and their target CpG sites. The red spikes show a master regulatory SNP rs12933229 located at 16p11.2 associated with methylation of CpG sites located in CGIs annotated to five genes. (b) Proportion of CpG probes detected withcis-meQTLs andtrans-meQTLs across gene regions. The asterisks ‘*, **, ***’ indicatet-testP<0.05, 0.01 and 0.0001, respectively, for the comparison between CGI and non-CGI regions. CGI regions are strongly enriched withtrans-meQTLs, while non-CGI regions are enriched withcis-meQTLs. CpG sites in 3′ UTR regions show an opposite trend. (c) The association between a SNP denoted as G and a distal CpG-site B may be mediated through a proximal CpG-site A. (d) For eachtrans-association (G,B) pair, the dots show their marginal versus partial correlation coefficients upon conditioning on the proximal A CpG probes. Analysis was based on 210 samples. Reduction of correlation coefficients by conditioning on A suggests the magnitude of the mediation effect. Figure 2: trans -meQTL structural characteristics. ( a ) Circos plot for trans -meQTLs. The outer rim shows the log 10 P -values Manhattan plots of trans -meQTL associations. The innermost network depicts spokes between all trans -meQTL SNPs and their target CpG sites. The red spikes show a master regulatory SNP rs12933229 located at 16p11.2 associated with methylation of CpG sites located in CGIs annotated to five genes. ( b ) Proportion of CpG probes detected with cis -meQTLs and trans -meQTLs across gene regions. The asterisks ‘*, **, ***’ indicate t -test P <0.05, 0.01 and 0.0001, respectively, for the comparison between CGI and non-CGI regions. CGI regions are strongly enriched with trans -meQTLs, while non-CGI regions are enriched with cis -meQTLs. CpG sites in 3′ UTR regions show an opposite trend. ( c ) The association between a SNP denoted as G and a distal CpG-site B may be mediated through a proximal CpG-site A. ( d ) For each trans -association ( G , B ) pair, the dots show their marginal versus partial correlation coefficients upon conditioning on the proximal A CpG probes. Analysis was based on 210 samples. Reduction of correlation coefficients by conditioning on A suggests the magnitude of the mediation effect. Full size image In 62.8% of the trans associations, the SNPs involved were also detected to have cis -acting effects. We investigated whether trans associations were mediated by these cis -regulated proximal CpG sites ( Fig. 2c,d ). We found that 30 and 166 trans associations had full and partial mediation, respectively, while 389 had no significant mediation. The trans associations involving SNPs in gene desert regions are less likely to be mediated by proximal CpG probes (15.7 versus 34.3%; P =0.0067, Fisher’s exact test). To obtain mechanistic insight into the trans associations showing mediation effects ( n =196), we used the DAVID tool [23] to characterize the function of genes harbouring the mediating cis -CpG probes. The analysis was performed for 115 genes after excluding the major histocompatibility complex (MHC) region because of long-range complex LD patterns. The GO analysis revealed three top gene categories with nominal significance involved in DNA methylation regulation, including GTPase-activity related genes ( P =0.004, Fisher’s exact test), genes regulating transcription ( P =0.02) and genetic imprinting ( P =0.04, Fisher’s exact test, Supplementary Table 2 ). Notably, 106 trans SNPs with P <2.5 × 10 −10 were associated with multiple distal CpG probes, suggesting that they are multi-CpG regulators. In particular, we detected one master regulatory SNP, rs12933229 located at 16p11.2, in a very large intron of the NPIPL1 gene, which was associated with the methylation of CpG sites annotated to five genes on different chromosomes ( Fig. 2a , Supplementary Fig. 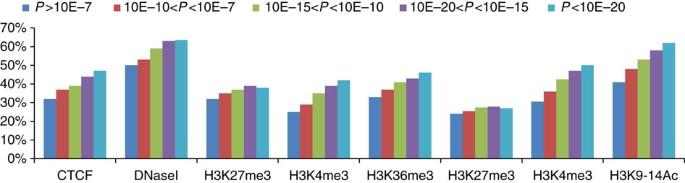Figure 3: Chromatin marks are increasingly enriched on meQTL SNPs with larger effect sizes. (a) We splitcis-meQTL SNPs into five categories according to the meQTL association strength (P>10−7, 10−7>P>10−10, 10−10>P>10−15, 10−15>P>10−20andP<10−20). A SNP is determined to be related with a regulatory region if the SNP or any LD-related SNP (r2≥0.8) resides in the ChIP-Seq peaks of the regulatory regions. Regulatory elements include CTCF-binding sites, DNaseI hypersensitive sites and histone marks from SAEC from ENCODE and hAEC from our laboratory. For eachP-value category, we calculated the proportions ofcis-meQTL SNPs related with regulatory regions. The figures show that the proportions ofcis-meQTL SNPs related with regulatory regions increase with the significance of meQTL associations except for the repressive mark H3K27me3. 2 and Supplementary Table 3 ). These associations were partially mediated by a proximal CpG probe cg06871736. All five trans associations were replicated in TCGA. The trans associations show a consistent direction, with the ‘C’ allele associated with higher methylation levels. All five regulated target sites are in CGIs, and three are in gene promoter regions. We evaluated the association with gene expression for these three CpG probes, using 28 TCGA histologically normal lung tissue samples with RNA sequencing data. Based on this limited sample size, two of the target genes, PABPC4 and STARD3 , showed decreased expression with increased methylation (FDR=10%). Enrichment of meQTLs in DNA regulatory regions SNPs associated with complex diseases in genome-wide association studies (GWAS) or with eQTLs have been reported to be enriched in ENCODE-annotated regulatory regions [24] , [25] . These include DNaseI hypersensitivity sites, CCTC-binding factor (CTCF) binding sites and regions enriched in active and repressive histone modification marks. The large number of meQTLs detected in our study, both cis and trans , enabled us to systematically investigate their enrichment in regulatory regions. We performed enrichment analysis using Chip-Seq data in small airway epithelial cells (SAEC) from the ENCODE project for histone marks [26] , CTCF occupancy [27] and DNaseI hypersensitivity sites [28] , and histone marks in primary human alveolar epithelial cells (hAEC) from our own laboratory [29] . Compared with the ‘control’ SNP set not associated with the methylation of CpG sites (with minor allele frequency (MAF) and CpG probe density matched with meQTL SNPs), the meQTL SNPs were strongly enriched for sites of CTCF, DNaseI hypersensitivity and histone marks (H3K4me3, H3K9-14Ac and H3K36me3) associated with active promoters, enhancers and active transcription, and to a lesser extent for the repressive mark H3K27me3 ( Table 2 ). Enrichment of all regulatory regions became stronger with increasing significance of association, with the exception of the H3K27me3 repressive mark ( Fig. 3 ). Using SAEC CTCF ChIP data, we found that meQTL SNPs or associated SNPs in high LD located within CTCF consensus sequences can affect allele-specific binding of CTCF (see two examples in Supplementary Figs 3 and 4 ). Table 2 Chromatin marks are enriched on meQTL SNPs. Full size table Figure 3: Chromatin marks are increasingly enriched on meQTL SNPs with larger effect sizes. ( a ) We split cis -meQTL SNPs into five categories according to the meQTL association strength ( P >10 −7 , 10 −7 > P >10 −10 , 10 −10 > P >10 −15 , 10 −15 > P >10 −20 and P <10 −20 ). A SNP is determined to be related with a regulatory region if the SNP or any LD-related SNP ( r 2 ≥0.8) resides in the ChIP-Seq peaks of the regulatory regions. Regulatory elements include CTCF-binding sites, DNaseI hypersensitive sites and histone marks from SAEC from ENCODE and hAEC from our laboratory. For each P -value category, we calculated the proportions of cis -meQTL SNPs related with regulatory regions. The figures show that the proportions of cis -meQTL SNPs related with regulatory regions increase with the significance of meQTL associations except for the repressive mark H3K27me3. Full size image Lung cancer risk SNPs affect methylation in human lung tissue To determine whether the identified meQTLs might provide functional annotation to the established genetic associations with lung cancer risks, we examined SNPs in five genomic regions reported to be associated with lung cancer risk in GWAS of populations of European ancestry: 15q25.1 (refs 30 , 31 , 32 ) ( CHRNA5–CHRNA3–CHRNB4 ), 5p15.33 (refs 20 , 33 , 34 ), 6p21.33 (ref. 33 ) ( BAT3 , most strongly associated with squamous cell carcinoma or SQ), 12p13.3 (ref. 35 ) ( RAD52 for SQ) and 9p21.3 (ref. 36 ) ( CDKN2A/CDKN2B, particularly for SQ). The GWAS SNPs at 15q25.1 were reported to be associated with total expression levels and multiple isoforms of CHRNA5 in normal lung tissue samples [37] , [38] . The GWAS SNPs at the other four loci have not been reported to be associated with the total expression of nearby genes. Consistently, we did not observe an association in RNA-seq data from TCGA lung normal tissue samples ( n =59), although a detailed investigation of alternative promoters, splice sites and allele-specific gene expression in larger studies is warranted. Here we investigated whether these SNPs contributed to lung cancer risk with epigenetic regulation by examining their associations with DNA methylation levels. The top GWAS SNPs located at 15q25.1, 5p15.33, 6p21.33 and 12p13.3 were all strongly associated with the methylation of the nearby CpG probes and the associations were replicated in TCGA lung data ( Fig. 4 ). Importantly, five of the six GWAS SNPs at these loci, excluding the RAD52 locus, were also the SNPs with the strongest association with the corresponding CpG probes. For the cg22937753 probe located in the RAD52 locus, another SNP, rs724709, with weak correlation with the GWAS SNP ( r 2 =0.1) had the strongest association with meQTL. All involved CpG sites are located within gene bodies (which may affect gene splicing [39] ) or the 3′UTR regions. No meQTL was detected for 9p21.3 ( Supplementary Fig. 5 ), possibly because of fewer CpG dinucleotide probes available in this gene region on the Illumina platform. The location of these lung cancer GWAS-associated CpG sites might identify which genes within the relevant regions are more likely associated with the risk SNPs, something that is particularly important for regions with complex LD structure, as the MHC region on 6p21. In MHC, two GWAS SNPs in complete LD ( r 2 =1), rs3117582 ( BAT3 ) and rs3131379 ( MSH5 ), were most strongly associated with the methylation of CpG sites located nearby of MSH5 (involved in DNA mismatch repair and meiotic recombination process), suggesting that MSH5 ( P =5.4 × 10 −13 , t -test) is more likely to be involved in lung carcinogenesis than BAT3 ( P =8.8 × 10 −5 , t -test) or that the SNP closer to MSH5 (rs3131379) is more likely to be the SNP most responsible of the GWAS association with lung cancer risk ( Fig. 4b ). Our meQTL data also show that rs3131379 trans -regulated the methylation level of CpG probe cg12093005, located in the body of FBRSL1 at 12q24 ( P EAGLE =4.0 × 10 −9 , P TCGA =7.2 × 10 −4 and P combined =5. 4 × 10 −11 , t -test). Thus, this known GWAS locus might affect lung cancer risk through a gene located on a different chromosome. 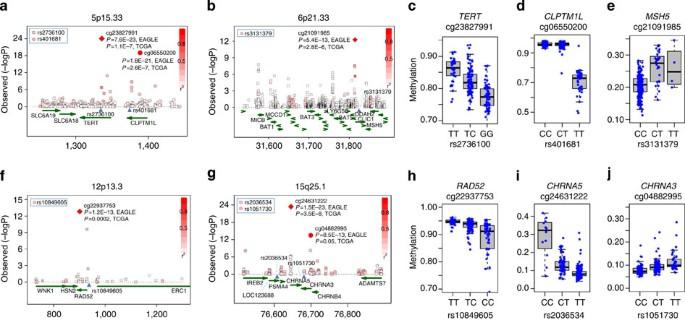Figure 4: DNA methylation regional associations for lung cancer GWAS SNPs in subjects of European ancestry. (a,b,f,g) Symbols represent the association between established lung cancer GWAS genetic loci in four regions and methylation levels in nearby CpG probes.ycoordinate,P-value for association;xcoordinate, genomic location. For each SNP, the red solid circle or square represents the methylation probe with the strongest association, whereas other methylation probes are coloured on the basis of their correlation (measured asr2) to the most-associated probe. For the most-associated probes, theP-values in EAGLE discovery set (n=210) and TCGA lung replication data (n=65) are shown. SNP locations are marked by a blue triangle. (c–eandh–j) show the associations between genotypes and methylation levels of the most-associated CpG probes. The box plots show the distribution of the methylation levels in each genotype category with error bars representing the 25 and 75% quantiles. Figure 4: DNA methylation regional associations for lung cancer GWAS SNPs in subjects of European ancestry. ( a , b , f , g ) Symbols represent the association between established lung cancer GWAS genetic loci in four regions and methylation levels in nearby CpG probes. y coordinate, P -value for association; x coordinate, genomic location. For each SNP, the red solid circle or square represents the methylation probe with the strongest association, whereas other methylation probes are coloured on the basis of their correlation (measured as r 2 ) to the most-associated probe. For the most-associated probes, the P -values in EAGLE discovery set ( n =210) and TCGA lung replication data ( n =65) are shown. SNP locations are marked by a blue triangle. ( c – e and h – j ) show the associations between genotypes and methylation levels of the most-associated CpG probes. The box plots show the distribution of the methylation levels in each genotype category with error bars representing the 25 and 75% quantiles. Full size image Of note, on the 15q25.1 locus, two independent lung cancer risk SNPs, rs2036534 and rs1051730, were associated with CpG probes not linked with CHRNA5 expression. In Supplementary Fig. 6 , we show that the two SNPs jointly regulated another methylation probe cg22563815 within the CHRNA5 promoter, which is associated with CHRNA5 expression. This extends and further confirms the complex regulatory pattern with multiple SNPs previously observed for this locus [35] . Most subjects in the analyses were smokers ( n =206). Adjustment for smoking status (former and current) or intensity (pack/years) did not change the results. cis -meQTLs are enriched in lung SQ risk We investigated whether the identified cis -meQTL SNPs were enriched in the National Cancer Institute (NCI) lung cancer GWAS including 5,739 cases and 5,848 controls of European ancestry [19] . To focus on potentially new genetic risk associations, we excluded the top lung cancer GWAS SNPs mentioned above and their surrounding regions. We tested the enrichment by examining whether the GWAS P -values for the LD-pruned cis -meQTL SNPs deviated from the uniform distribution, that is, no enrichment. When all cis -meQTL SNPs were analysed together, we detected a strong enrichment for overall lung cancer risk ( P <10 −4 , based on 10,000 permutations), which was primarily driven by the enrichment in SQ ( P <10 −4 , based on 10,000 permutations) ( Fig. 5a ). The genomic control λ values based on genome-wide SNPs showed that the type-I error rates of our enrichment test were not inflated ( λ =1.01 and 1.00, for overall lung cancer and SQ, respectively). Stratified analyses further refined the enrichment to the cis -meQTL SNPs regulating CpG sites mapping to north shore ( Fig. 5b ) and gene body ( Fig. 5c ) regions (see Supplementary Fig. 7 for the quantile–quantile plot). These gene bodies and north shores were enriched for genes involved in cancer pathways ( P =2.5 × 10 −4 , Fisher’s exact test), and particularly those in NSCLC pathway (for example, AKT1 , MAPK1 , RASSF5 , and so on, Supplementary Table 4 ). In contrast, cis -meQTLs related with CGI regions or promoters were not enriched with the risk of overall lung cancer or any lung cancer subtype, further emphasizing the need to comprehensively study the methylome to identify functional mechanisms for GWAS findings and identify new genetic loci. 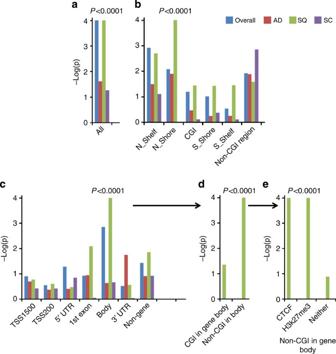Figure 5: Enrichment ofcis-meQTL SNPs for lung cancer risk. Analysis based on NCI lung cancer GWAS data (5,739 cases and 5,848 controls).P-values were produced based on 10,000 permutations. AD, SQ and SC represent adenocarcinoma, squamous cell carcinoma and small cell carcinoma. (a) Enrichment was tested using allcis-meQTL SNPs after LD pruning. (b,c) Strong enrichments were observed forcis-meQTL SNP associated with CpG probes annotated to north shores (b) and gene body (c) regions for SQ. (d) The enrichment in (c) was driven by thecis-meQTLs SNPs impacting CpG probes in non-CpG islands. (e) The enrichment in (d) is driven by the SNPs (or their LD SNPs withr2>0.95) overlapping with CTCF binding sites or H3K27me3 mark regions. Figure 5: Enrichment of cis -meQTL SNPs for lung cancer risk. Analysis based on NCI lung cancer GWAS data (5,739 cases and 5,848 controls). P -values were produced based on 10,000 permutations. AD, SQ and SC represent adenocarcinoma, squamous cell carcinoma and small cell carcinoma. ( a ) Enrichment was tested using all cis -meQTL SNPs after LD pruning. ( b , c ) Strong enrichments were observed for cis -meQTL SNP associated with CpG probes annotated to north shores ( b ) and gene body ( c ) regions for SQ. ( d ) The enrichment in ( c ) was driven by the cis -meQTLs SNPs impacting CpG probes in non-CpG islands. ( e ) The enrichment in ( d ) is driven by the SNPs (or their LD SNPs with r 2 >0.95) overlapping with CTCF binding sites or H3K27me3 mark regions. Full size image As the meQTL SNPs affecting CpG sites in gene body/non-CGI regions were mostly enriched for SQ risk ( Fig. 5d ), we performed further analysis in this category by integrating the ENCODE SAEC data. We chose SAEC data because this cell type may be involved in SQ development. We restricted enrichment analysis to the ‘regulatory’ meQTL SNPs, which localized in the CTCF binding regions, DNaseI hypersensitive sites or histone marks (H3K27me3, H3K4me3 and H3K36me3) or had at least one LD SNP ( r 2 ≥0.95) residing in these regions. The strong enrichment in SQ was driven by SNPs overlapping with CTCF binding sites ( P <10 −4 , based on 10,000 permutations) or the repressive mark H3K27me3 ( P <10 −4 , based on 10,000 permutations) ( Fig. 5e ). The enrichment test was not significant after excluding the SNPs overlapping with these regulatory regions ( P =0.14, based on 10,000 permutations). Replication of meQTLs in TCGA breast and kidney tissues To explore the tissue specificity of the genetic effects on DNA methylation, we examined whether the meQTLs detected in EAGLE lung tissue data could be replicated in TCGA breast ( n =87) or kidney ( n =142) histologically normal tissue samples, the only two organs to date with data available for a large number of normal tissues of European ancestry. Results are provided in Table 1 and Supplementary Fig. 8 . For both cis - and trans -meQTLs, a large proportion of associations had the same direction of EAGLE meQTLs in both breast and kidney samples. For cis associations, 54.7 and 70.0% were replicated with FDR=5% based on single-sided P -values in two data sets, respectively. For the strong cis associations with P <10 −10 in EAGLE, the replication rates increased to 82.7 and 89.2% in the two data sets. For trans associations, 83.4 and 86.4% were replicated in breast and kidney samples, respectively. The detected master regulator ( Fig. 2a ) was strongly replicated in both data sets ( Supplementary Table 3 ). Interestingly, some cis -meQTLs, but not trans -meQTLs, had an opposite but very strong association ( P <10 −6 ) in breast ( n =7) or kidney ( n =58) compared with the EAGLE lung data, a phenomenon previously reported in a cell type-specific eQTL study [40] . We found that inherited genetic variation profoundly and extensively impacts DNA methylation in target organs. Based on high-density methylation arrays in a large sample size, we identified 34,304 cis -meQTLs and 585 trans -meQTLs, one to two orders of magnitude larger compared with previous studies [3] , [4] , [5] , [7] . meQTLs involved nearly half of the autosomal genes, of which 9,330 in cis and 373 in trans , with 9,525 unique genes in total. We show that ~10% of the cis -meQTLs were affected by at least two SNPs independently. Moreover, we detected a master regulator SNP associated with the methylation levels of five CpG probes on different chromosomes, demonstrating the existence of regulatory hotspots for DNA methylation, as previously shown for eQTL [41] , [42] . Most meQTLs were replicated in independent histologically normal lung tissue samples from TCGA. We also showed a high similarity of genetic control on DNA methylation across different tissues. Our findings show that genetic effects on DNA methylation are extensive in scale and complex in structure across the whole genome and suggest a series of important biological implications. First, our results show that the genomic architecture surrounding cis - and trans -meQTLs is distinct. cis -meQTLs are very large in number, impact predominantly the CpG sites mapping to non-gene regions, and when they occur in genes, are mostly in non-promoter and non-CpG island regions. In contrast, trans -meQTLs are rarer, mainly affect promoter CGI regions, and may be associated with distal CpG sites through the mediation effect of proximal CpG sites. We found preliminary evidence that the cis -CpG sites mediating the trans -meQTL associations were enriched for genes involved in methylation regulation, such as genes encoding for GTPase or proteins involved in genetic imprinting. GTPase-related gene pathways appear to modulate expression of DNA methyltransferases [43] . Methylation-induced expression changes of these genes may result in further methylation changes of other genes (that is, in trans ). Moreover, a noncoding RNA within the intron of KCNQ1 , a key gene regulating genetic imprinting, can influence chromatin three-dimensional (3D) structure via a protein complex including DNA methyltransferase proteins [44] , [45] . These findings suggest intricate mechanisms for trans -regulating effects through proximal methylation. cis -meQTLs may affect cancer risk. To understand the functional consequences of GWAS loci is challenging and multiple principles for post-GWAS’ functional characterization of genetic loci have been proposed, including the exploration of epigenetic mechanisms [46] . In our study, the top GWAS lung cancer loci were strongly associated with methylation levels of CpG sites in nearby gene bodies through cis -regulation, and adjusting for smoking status or intensity did not change the results. Furthermore, SNPs affecting the DNA methylation of gene bodies (which are typically methylated) were also collectively associated with the risk for SQ after excluding the established GWAS loci, and were enriched for genes in cancer pathways. In contrast, no enrichment was observed for SNPs affecting the methylation of gene promoters or CGI regions, which are typically not methylated in normal tissues. This suggests a potential novel mechanism for genetic effects on cancer risk. In fact, gene body-enriched cis -meQTLs outside CGI regions may increase the risk for germline and somatic mutations due to their increased propensity to become mutated [11] , [12] . Upon spontaneous hydrolytic deamination, methylated cytosine residues turn into thymine, which are less likely to be efficiently repaired than the uracils that result from deamination of unmethylated cytosine residues. For example, ~25% of mutations in TP53 in cancers are thought to be due to epigenetic effects [47] . Indeed, analyses of comprehensive human catalogues of lung tumours have identified frequent G>T mutations enriched for CpG dinucleotides outside CGI regions, suggesting a role for methylated cytosine since CGI, as we confirmed, are usually unmethylated [48] . A similar signature was recently observed in other tumours [14] . Thus, inherited genetic variation may have a profound impact on carcinogenesis by regulating the human methylome. We observed a high similarity of genetic control on DNA methylation across tissues. Since tissue of origin determines cancer-associated CpG island promoter hypermethylation patterns [49] , a natural question is whether the genetic regulation of methylation is tissue-specific. While the tissue specificity of eQTLs has been investigated for a few tissues [50] , for cis -meQTL only a recent investigation was conducted [6] , showing that 35.7% of 88,751 cis -meQTLs detected in 662 adipose samples were replicated in ~200 whole-blood samples. We found that a large proportion of meQTLs in EAGLE lung samples, particularly those with large effect sizes, were robustly replicated in breast and kidney tissue samples from TCGA, suggesting a high similarity of genetic regulation of methylation across these tissues and related impact on somatic mutation rates [14] , [48] . The lower replication rate of adipose meQTLs in whole-blood samples [6] might be explained by the heterogeneity of different cell types in whole blood and by their more liberal P -value threshold (8.6 × 10 −4 ), which led to the identification of a large number of weak cis -meQTLs. Compared with cis -regulation, trans- eQTL regulation is typically considered to be more complex, has smaller effect sizes and is more difficult to be replicated even in the same tissue. However, in our study the lung trans -meQTLs are highly reproducible in TCGA lung, breast and kidney tissues. Notably, this similarity allows mapping meQTLs with substantially improved power by borrowing strength across tissues [51] . meQTL SNPs are strongly associated with multiple epigenetic marks. Chromatin regulators play a role in maintaining genomic integrity and organization [52] . We found that meQTL SNPs were strongly enriched for DNase hypersensitive sites, and sequences bound by CTCF or modified histones. SNPs could affect these epigenetic marks by several mechanisms, such as by affecting the core recognition sequences (exemplified for rs2816057 on chromosome 1 for CTCF), causing loss or gain of a CpG within a binding region, which, when methylated, could affect binding [27] , or altering the binding sequence for interacting factors [53] . CTCF could cause changes in epigenetic marks through its multiple key roles, including genome organization through mediating intra- and inter-chromosomal contacts [54] , [55] , the regulation of transcription by binding between enhancers and promoters [54] , [56] , and the regulation of splicing, which may impact tissue specificity during tissue development [39] . These changes can impact regulation of distant genes, and not the genes proximal to the SNPs that would be typically investigated in eQTL studies. This may be one reason for the previously observed lack of correlation between eQTLs and meQTLs [3] , [4] , [7] . Future large studies integrating SNP profiles, the DNA methylome and transcriptome data through tissue developmental stages will hopefully shed light on this possibility. There may be a myriad of other DNA-binding factors whose binding is directly or indirectly affected by SNPs. For example, among the histone marks, the strongest enrichment of meQTLs in our study was for H3K4me3 in both SAEC and hAEC cell types. As H3K4me3 is the chromatin mark primarily associated with regulatory elements at promoters, this suggests a strong influence of meQTLs on regulating gene activity. Unfortunately, transcription factor binding data in SAEC or hAEC are not available, so we could not test whether SNPs in their core sequence could affect the deposition of epigenetic marks, for example, by recruiting DNA methyltransferases [57] . It will be important to obtain ChIP data from relevant primary cells for numerous DNA-binding regulatory factors to further elucidate the mechanisms whereby meQTLs and other SNP-affected epigenetic marks arise. In conclusion, we show here that genetic variation has a profound impact on the DNA methylome with implications for cancer risk, tissue specificity, and chromatin structure and organization. The meQTL data ( Supplementary Data 1 and 2 ) attached to this manuscript provide an important resource for studying genetic–DNA methylation interactions in lung tissue. Sample collection We assayed 244 fresh-frozen paired tumour and non-involved lung tissue samples from Stage I to IIIA non-small cell lung cancer (NSCLC) cases from the EAGLE study [18] . EAGLE includes 2,100 incident lung cancer cases and 2,120 population controls enrolled in 2002–2005 within 216 municipalities of the Lombardy region of Italy. Cases were newly diagnosed primary cancers of lung, trachea and bronchus, verified by tissue pathology (67.0%), cytology (28.0%) or review of clinical records (5.0%). They were 35–79 years of age at diagnosis and were recruited from 13 hospitals that cover >80% of the lung cancer cases from the study area. The study was approved by local and NCI Institutional Review Boards, and all participants signed an informed consent form. Lung tissue samples were snap-frozen in liquid nitrogen within 20 min of surgical resection. Surgeons and pathologists were together in the surgery room at the time of resection and sample collection to ensure correct sampling of tissue from the tumour, the area adjacent to the tumour and an additional area distant from the tumour (1–5 cm). The precise site of tissue sampling was indicated on a lung drawing and the pathologists classified the samples as tumour, adjacent lung tissue and distant non-involved lung tissue. For the current study, we used lung tissue sampled from an area distant from the tumour to reduce the potential effects of field cancerization. DNA methylation profiling and data quality control Fresh-frozen lung tissue samples remained frozen while ~30 mg was subsampled for DNA extraction into pre-chilled 2.0 ml microcentrifuge tubes. Lysates for DNA extraction were generated by incubating 30 mg of tissue in 1 ml of 0.2 mg ml −1 Proteinase K (Ambion) in DNA Lysis Buffer (10 mM Tris–Cl (pH 8.0), 0.1 M EDTA (pH 8.0) and 0.5% ( w / v ) SDS) for 24 h at 56 °C with shaking at 850 r.p.m. in Thermomixer R (Eppendorf). DNA was extracted from the generated lysate using the QIAamp DNA Blood Maxi Kit (Qiagen) according to the manufacturer’s protocol. Bisulphite treatment and Illumina Infinium HumanMethylation450 BeadChip assays were performed by the Southern California Genotyping Consortium at the University of California Los Angeles (UCLA) following Illumina’s protocols. This assay generates DNA methylation data for 485,512 cytosine targets (482,421 CpG and 3091 CpH) and 65 SNP probes for the purpose of data quality control. Raw methylated and unmethylated intensities were background-corrected, and dye-bias-equalized, to correct for technical variation in signal between arrays. For background correction, we applied a normal-exponential convolution, using the intensity of the Infinium I probes in the channel opposite their design to measure non-specific signal [58] . Dye-bias equalization used a global scaling factor computed from the ratio of the average red and green fluorescing normalization control probes. Both methods were conducted using the methylumi package in Bioconductor version 2.11. For each probe, DNA methylation level is summarized as a β value, estimated as the fraction of signal intensity obtained from the methylated beads over the total signal intensity. Probes with detection P -values of >0.05 were considered not significantly different from background noise and were labelled as missing. Methylation probes were excluded from meQTL analysis if any of the following criteria was met: on X/Y chromosome, annotated in repetitive genomic regions, annotated to harbour SNPs and missing rate >5%. As the β values for the 65 SNP probes are expected to be similar in matched pair of normal and tumour tissues, we performed PCA using these 65 SNP probes to confirm the labelled pairs. We then performed PCA using the 5000 most variable methylation probes with var >0.02 and found that the normal tissues were clustered together and well separated from the tumour tissues. We further excluded five normal tissues that were relatively close to the tumour cluster. From the remaining 239 normal tissue samples, we analysed 210 with genotype data from a previous GWAS of lung cancer [20] . Genotype data and genetic association analysis The blood samples were genotyped using the Illumina HumanHap550K SNP arrays in EAGLE GWAS [20] . The SNPs with call rate >99%, MAF >3% and Hardy–Weinberg equilibrium P -value >10 −5 were included for analysis. Prior to meQTL analysis, each methylation trait was regressed against sex, age, batches and PCA scores based on methylation profiles. The regression residues were then quantile-normalized to the standard normal distribution N (0,1) as traits. The genetic association testing was performed using PLINK and R, adjusted for the top three PCA scores based on GWAS SNPs to control for potential population stratification. Identification of cis -meQTLs For each CpG methylation probe, the cis region was defined as being <500 kb upstream and downstream from the target CpG-site (1 Mb total). A methylation trait was detected to harbour a cis -meQTL if any SNP in the cis region had a SNP–CpG nominal association P -value less than P 0 , where P 0 was chosen to control FDR at 5% by permutations. Here we describe a permutation procedure to choose P 0 to control FDR at 5%. For a given P 0 , let N ( P 0 ) be the total number of CpG probes with detected cis -meQTLs and N 0 ( P 0 ) the expected number of CpG probes falsely determined to have cis -meQTLs. FDR is defined as N 0 ( P 0 )/ N ( P 0 ). The key is to estimate N 0 ( P 0 ) under the global null hypothesis that no CpG probe has cis -meQTLs. We randomly permuted the genotypes across subjects for 100 times, keeping the correlation structure of the 338,456 methylation traits in each permutation. Then, N 0 ( P 0 ) was estimated as the average number of methylation traits that were detected to harbour cis -meQTL SNPs with nominal P < P 0 . Control FDR at 5% requires P 0 =4.0 × 10 −5 . The same procedure was applied to detect secondary independently associated cis -meQTL SNPs. With our sample size, h 2 >0.12 is required to detect cis -meQTLs with power >0.8. We note that, although we excluded all CpG probes annotated with SNPs, there is still the possibility that rare, not annotated variants could be associated with the cis -meQTL SNPs. However, since common variants and rare variants are known to be poorly correlated, and rare variants are uncommon by definition, we do not expect this event to be frequent. Identification of trans -meQTLs For each CpG probe, the trans region was defined as being more than 500 kb from the target CpG site in the same chromosome or on different chromosomes. For the k th methylation trait with m SNPs in the trans region, let ( q k1 , ⋯ , q km ) be the P -values for testing the marginal association between the trait and the m SNPs. Let p k =min( q k1 , ⋯ , q km ) be the minimum P -value for m SNPs and converted p k into genome-wide P -value P k by performing one million permutations for SNPs in the trans region. As a cis region is very short (~1 M) compared with the whole genome (~3,000 M), P k computed based on SNPs in trans regions is very close to that based on permutations using genome-wide SNPs. Thus, we use the genome-wide P -value computed based on all SNPs to approximate P k . Furthermore, all quantile-normalized traits follow the same standard normal distribution N (0,1); thus the permutation-based null distributions are the same for all traits. We then applied the Benjamini–Hochberg procedure to ( P 1 , ⋯ , P N ) to identify trans -meQTLs by controlling FDR at 5%. With our sample size, h 2 >0.24 is required to detect trans -meQTLs with power >0.8. Replication of meQTLs in TCGA samples The replication was performed in TCGA histologically normal tissue samples that had genome-wide genotype (Affymetrix Genome-Wide Human SNP Array 6.0) and methylation profiling (Illumina Infinium HumanMethylation450 BeadChip). We downloaded genotype (level 2) and methylation data (level 3) from the TCGA website [22] . We also downloaded methylation data for tumour tissue samples and performed PCA analysis to confirm that normal tissue samples were separated from tumour tissue samples. Autosomal SNPs with MAF >3%, calling rate >0.99 and Hardy–Weinberg equilibrium P -value >10 −5 were included for imputation using IMPUTE2 (ref. 59) [59] and reference haplotypes in the 1,000 Genome Project [60] (version 2012/03). We only included samples of European ancestry based on EIGENSTRAT analysis. The replication set had 65 lung, 87 breast and 142 kidney histologically normal tissue samples after QC. Again, each methylation trait was regressed against sex, age, batches and PCA scores based on methylation profiles. The regression residues were then quantile-normalized to the standard normal distribution N (0,1) as traits for meQTL analysis. The associations were tested between the quantile-normalized methylation traits and imputed genotypic dosages, adjusting for sex, age and PCA scores based on SNPs. A genetic association detected in EAGLE lung data was considered replicated if the association had the same direction and FDR <0.05 based on single-sided P -values. Testing genetic associations with methylation and gene expression traits We downloaded gene expression data (level 3) from RNA-seq analysis of 59 histologically normal tissue samples from NSCL patients from TCGA. All samples also had genome-wide genotype data, and 28 samples had additional methylation data from Illumina Infinium HumanMethylation450 BeadChips. Regression analysis was performed to test the association of gene expression with methylation levels in the CHRNA5 gene and with methylation levels in PABPC4 , STARD3 and SLC35A3 genes. We tested the association between lung cancer GWAS risk SNPs and gene expression using regression analysis under an additive model, adjusting for age, sex and PCA scores based on genome-wide SNPs. Testing for enrichment of cis -meQTLs in lung cancer GWAS We tested for enrichment in NCI lung cancer GWAS of European ancestry, which included three main histologic subtypes of lung cancer (adenocarcinoma (AD), SQ, small cell carcinoma (SC)) and a small number of other lung cancer subtypes. We investigated whether the identified cis -meQTL SNPs were collectively associated with lung cancer risk, which was tested by examining whether the GWAS P -values for these SNPs deviated from the uniform distribution (that is, no enrichment). As the high LD in SNPs increased variability of the enrichment statistic and caused a loss of power, we first performed LD pruning using PLINK so that no pair of remaining SNPs had an r 2 ≥0.8. The enrichment significance was evaluated by 10,000 random permutations. The genomic control λ values [61] based on genome-wide SNPs were 1.01, 0.995, 0.977 and 1.00 for overall lung cancer, AD, SC and SQ, respectively. Thus, the type-I error rates of our enrichment tests were not inflated. The detailed procedure for testing a set of cis -meQTL SNPs is described as follows: First, we performed LD-pruning using PLINK so that no pair of remaining SNPs had an r 2 ≥0.8. Second, we tested the association for the LD-pruned SNPs (assuming K SNPs left) in a GWAS and computed the P -values ( p 1 , ⋯ , p K ). We then tested whether ( p 1 , ⋯ , p K ) followed a uniform distribution, that is no enrichment. Third, we transformed P -values into quantitles with being the cumulative distribution function (CDF) of . We defined a statistic for testing enrichment as [35] , [62] , where f is a pre-specified constant reflecting the expected proportion of SNPs associated with the disease. As only a small proportion of SNPs may be associated with the disease, we set f =0.05 for this paper. The statistical power was insensitive to the choice of f in the range of [0.01, 0.1] [62] . Finally, the significance of the test Q was evaluated by 10,000 random permutations. meQTL mediation analysis We investigated whether trans associations were mediated by the methylation levels of CpG probes nearby the trans -acting SNPs. Note that this analysis was only for trans associations with cis effects, that is, the SNP was associated with at least one proximal CpG probes with P <4 × 10 −5 . See Fig. 2c . Suppose an SNP G cis -regulates K proximal (<500 kb) CpG sites A 1 , ⋯ , A K with P <4 × 10 −5 and trans -regulates a distal CpG site B . We performed a linear regression: B~α+θG +λ k A k . We also computed marginal correlation coefficient cor ( G , B ) and partial correlation coefficient cor ( G , B|A k ) using an R package ‘ppcor’ [63] . A full mediation was detected if G and B were not significantly correlated after conditioning on A k , or equivalently G was not significant ( P >0.01) in regression analysis B~α+θG +λ k A k for any k . A partial mediation was detected if any A k had a P<0.05/K (Bonferroni correction) in the regression analysis and |cor( G , B ) |−| cor( G , B|A ) |>0.1. An independent effect model (that is, no mediation) was detected otherwise. Testing enrichment of meQTL SNPs in regulatory regions We obtained peak data for CTCF, DNaseI, H3K27me3, H3K4me3 and H3K36me of SAEC from the ENCODE project and for H3K27me3, H3K4me3 and H3K9-14Ac from hAEC from our own laboratory. A SNP is determined to be functionally related to a given mark or CTCF binding site if the SNP or any of its LD SNPs ( r 2 ≥0.8 with LD computed using the genotype data of European population in The 1000 Genome Project) resided in any of the mark regions or CTCF binding sites. We explain our enrichment testing using CTCF as an example. We classified genome-wide SNPs into four categories: SNPs not associated with CpG probes in trans or cis (defined as control SNP set), SNPs only associated with proximal CpG probes via cis -regulation ( cis -only, 21,119 SNPs), SNPs only associated with distal CpG probes via trans -regulation ( trans -only, 192 SNPs) and SNPs detected with both trans and cis effects ( cis + trans , 277 SNPs). For SNPs in the category of cis -only, trans -only and cis + trans , we computed the proportion of SNPs functionally related to CTCF. To compute the enrichment of cis -meQTLs in CTCF binding sites, we defined a control set of SNPs that are not associated with CpG probes via cis - or trans regulation. The selection of the control set was further complicated by the following two observations. (1) cis -meQTL SNPs tended to be more common (data now shown). (2) The probability of a SNP detected as a cis -meQTL SNP positively depended on the density of the CpG probes in the nearby region. Choosing a control set while ignoring these two factors could underestimate the proportion of functionally related SNPs in the control set and thus overestimate the enrichment for cis -meQTLs. Therefore, we created 1,000 sets of control SNPs with CpG probe density (measured as the number of CpG probes in the cis region of each SNP) and MAF matched with the meQTL SNP set, and then averaged the proportions on the 1,000 sets. The enrichment was calculated as the fold change with the proportion in the control SNP set as baseline. Next, we investigated whether the enrichment was stronger for SNPs more significantly associated with CpG sites. As we detected only a few hundred trans -meQTLs, we focused this analysis on the set of cis -meQTLs. We classified cis -meQTL SNPs into five categories according to the cis -association P -values: P >10 −7 (the weakest), 10 −10 < P ≤10 −7 , 10 −15 < P ≤10 −10 , 10 −20 < P ≤10 −15 and P ≤10 −20 (the strongest). For each category, we computed the proportion of SNPs functionally related to CTCF-binding sites. meQTL SNPs affect CTCF binding We found that meQTL SNPs are strongly enriched in CTCF consensus sequences. We used SAEC data from ENCODE to test whether meQTL heterozygous SNPs directly affect CTCF binding by disrupting the CTCF recognition sites. P -values were calculated based on a binomial distribution Binom( N , 0.5). Here N is the total number reads covering the SNPs. Raw sequencing data (.fasstq format) from SAEC cells were generated at the University of Washington as part of the ENCODE project and downloaded from the UCSC genome browser. Raw data was aligned to the hg19 genome using CLC genomics workbench (v 5.5.1), parsing out data with <80% contiguous alignment to the genome and duplicate reads in excess of 10 copies. We used the CTCFBSDB 2.0 programme [64] to predict whether the meQTL SNPs or their LD SNPs ( r 2 ≥0.8) were within CTCF peaks and then examined in SAEC whether CTCF exhibited allele-specific binding. As common SNPs are more likely to be heterozygous, we only looked for SNPs with MAF ≥0.4. Here we present two such examples. Systematic investigation of all meQTL SNPs that are heterozygous in SAEC is warranted once more samples with genotypic data are available. Accession codes: Genotype data have been deposited in dbGAP under accession code phs000093.v2.p2. Methylation data have been deposited in dbGAP under accession code GSE52401. How to cite this article: Shi, J. et al. Characterizing the genetic basis of methylome diversity in histologically normal human lung tissue. Nat. Commun. 5:3365 doi: 10.1038/ncomms4365 (2014).